Subcellularin vivotime-lapse imaging and optical manipulation ofCaenorhabditis elegansin standard multiwell plates High-resolution in vivo time-lapse assays require repeated immobilization and imaging of whole animals. Here we report a technology for screening Caenorhabditis elegans at cellular resolution over its entire lifespan inside standard multiwell plates using repeated immobilization, imaging and optical manipulation. Our system does not use any fluidic or mechanical components, and can operate for tens of thousands of cycles without failure. It is also compatible with industrial high-throughput screening platforms and robotics, and it allows both chemical, and forward and reverse genetic screens. We used this technology to perform subcellular-resolution femtosecond laser microsurgery of single neurons in vivo , and to image the subsequent regeneration dynamics at subcellular resolution. Our single-neuron in vivo time-lapse analysis shows that neurite regrowth occurring over short time windows is significantly greater than that predicted by ensemble averaging over many animals. High-throughput screening (HTS) allows rapid identification of potential therapeutic targets and leads. Although high-throughput assays can be performed in vitro , thorough study of many biological phenomena, such as development, organogenesis, regeneration and aging, requires the use of animal models. The use of multicellular organisms also facilitates identification of off-target or toxic effects. The nematode Caenorhabditis elegans is one of the most commonly used multicellular organisms for HTS. As nematodes can be cultured and screened in liquid, many techniques currently used for screening cells can be adapted for C . elegans . The small size and simple physiology of C . elegans render it suitable for culture in 96- and 384-well plates in small volumes, and internal organs can be easily visualized because C. elegans is optically transparent. Investigation of C. elegans often involves high-content and time-lapse studies; however, these rapidly moving organisms must be immobilized to image cellular and subcellular processes. In addition, many physiological processes are stochastic and time-dependent (that is, development, aging), which requires multitime-point immobilization, tracking, and imaging of large numbers of individual animals. Commercially available technologies for HTS of C. elegans utilize flow cytometry [1] , [2] , [3] . Despite their speed, these systems can acquire only one-dimensional fluorescence images. Thus, assays requiring analysis of cellular and subcellular features are not feasible. In addition, optical measurements and manipulations, such as multiphoton [4] and confocal imaging, laser stimulation and laser microsurgery [5] , [6] , [7] , are not possible with such approaches. Recently, we and others developed microfluidic approaches for immobilization of C. elegans for high-throughput and high-content screening. Mechanical immobilization (both active [8] , [9] , [10] , [11] and passive [12] ) and cooling [13] have been used to enable short-term immobilization. Three-dimensional multiphoton imaging [9] , [10] and femtosecond laser microsurgery [9] , [10] , [11] have both been demonstrated in some of these devices. We also previously demonstrated multiplexed microfluidic chambers for long-term incubation, immobilization and imaging of C. elegans [8] . Other approaches since then have used CO 2 [14] , tapered channels [15] or temperature-sensitive gel [16] combined with microfluidics to enable longer-term time-lapse imaging of animals. Despite their capabilities, these microfluidic systems are still too complex to manufacture, operate, maintain and scale for mainstream use. Integration of these techniques into existing HTS platforms in order to enable delivery of library compounds to C. elegans incubated on-chip has been challenging because of the well-known 'world-to-chip' fluidic interface issues [17] . Although C. elegans can be anaesthetized in HTS-compatible multiwell plates for immobilization and imaging, the effects of anaesthesia are slow and variable and removal of the anaesthetic media without losing animals is highly unreliable. In addition, exposure to anaesthetics has side effects [18] . We recently demonstrated the use of multiwell plates with microfluidics to enable incubation of large numbers of C. elegans in chemical libraries, following femtosecond laser microsurgery inside microfluidic chips [19] . Although this offered a partial solution to the problem of interfacing with HTS platforms, the complexity involved in manufacturing and running such specialized microfluidic devices has remained a major obstacle for widespread use. Here we demonstrate a simple method to rapidly image and optically manipulate C. elegans at subcellular resolution in standard multiwell plates at multiple time points by modulating the temperature of individual wells. Our method is fully compatible with existing instruments, robotics and protocols used in industrial HTS platforms. Furthermore, our system does not use any fluidic or mechanical components, and can operate for tens of thousands of cycles without failure. It can perform both chemical, and forward and reverse genetic screens at cellular resolution in vivo . In total, only a few minutes are needed to immobilize the animals when screening an entire plate, and animals are immobilized only during the brief period in which they are imaged, thus minimizing stress. Our technology can significantly accelerate most C. elegans investigations. Our immobilization technique also enables the use of subcellular-precision optical manipulation methods such as femtosecond laser microsurgery [5] , [6] , [7] . We have previously shown the use of femtosecond laser microsurgery to study regeneration in C. elegans [5] , [6] . Here, we show the use of our new immobilization technique to study the time-dependent regeneration dynamics of single neurons after in vivo femtosecond laser microsurgery in standard multiwell plates. Our single-neuron in vivo time-lapse analysis shows that neurite regrowth occurring over short time windows is greater than that predicted by ensemble averaging over many animals. In-well cooling apparatus and its operation It is well known that cooling reduces the motion of C. elegans [20] . Our device consists of an array of individually addressable cooling elements that rapidly modulate the temperature of each well independently. Each individual cooling element consists of a small square thermoelectric cooler (TEC) bonded to an aluminium pin (which is inserted into the well) and a copper pin (which is used to dissipate heat; Fig. 1a ). The copper pins of the individual cooling elements are slotted into a copper backplane that is passively cooled, and the individual pins are inserted into the wells ( Fig. 1b ). This design is easily scalable to different well numbers and dimensions. Independent control of well temperatures allows much faster screening of wells by pipelining: While animals in one well are being imaged using inverted epi-fluorescence microscopy, the neighbouring wells that have yet to be imaged can be gradually cooled to immobilize the animals in preparation for subsequent imaging and optical manipulation ( Fig. 1c ), which completely eliminates the time required for cooling and immobilization ( Fig. 1e ). Once the animals within the first well are imaged, the cooling element is immediately turned off, allowing the animals to return to room temperature while the already-cooled animals in the next well are imaged. This prevents the animals from being exposed to low temperatures over the entire duration for which the multiwell plate is imaged. During the cooling period, the temperature of the wells reaches 3–4 °C, with little cooling of the adjacent wells ( Fig. 1d ) and negligible cooling of the wells beyond these. At the centre of the adjacent wells, the temperature stays above 16 °C (even after prolonged cooling), which is within the normal temperature range used for C. elegans culture. A temperature of 3–4 °C was found to be the threshold temperature required to immobilize C. elegans ; higher temperatures did not sufficiently slow the animals' movement. On average, <20 s (thus ∼ 32 min per plate) is required for all steps needed to image animals in the subsequent wells, including the time required to locate the animal, move the multiwell plate to centre the animal within the field of view, change objectives for high-resolution imaging, store images and switch back to a low-magnification objective ( Fig. 1e ). Following screening, the pins can be sterilized via heating by running the TEC in reverse ( Supplementary Fig. S1 ). 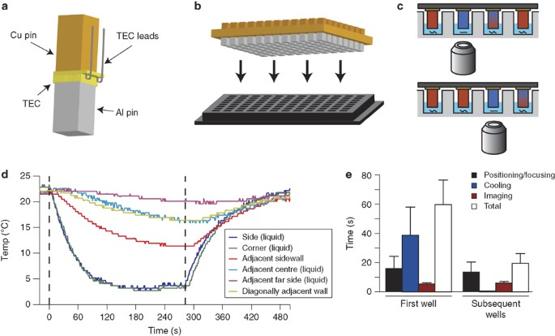Figure 1: Design and characterization of the in-well cooling system. (a–c) In-well cooling device and its operation. (a) Individual cooling elements consist of an aluminium pin bonded to a thermoelectric cooler (TEC) with a copper pin bonded to the opposite side to dissipate heat. (b) Cooling elements can be arrayed to match various well configurations. (c) Pipelined cooling. Thermoelectrically cooled pins are inserted into wells containing animals. Once activated, a cooling element reduces the temperature of the well, immobilizing the animal(s) within that well. Immobilized animals are imaged or optically manipulated using inverted epifluoresence microscopy. Concurrently, neighbouring wells are cooled such that the animals to be subsequently imaged are immobilized in advance. (d) Temporal and spatial dependency of the temperature inside the well being cooled (near the sides and corners), in an orthogonally adjacent well (near the wall adjacent to the well being cooled, near the adjacent-well centre and near the side of adjacent well that is furthest from the well being cooled) and in a diagonally adjacent well (near the corner closest to the well being cooled). Thermoelectric cooling was started att=0 s (first dashed line) and stopped att=280 s (second dashed line). SeeMethodsfor measurement technique. (e) Time required for imaging animals inside a well plate with a single animal per well. Following imaging of the first animal in the well (n=20), pipelined cooling enables much faster imaging of the subsequent animals (n=95). The time reported for positioning/focusing includes the time required to move the position stage from well to well, locate an animal using a ×2 objective lens, switch to a ×20 objective lens and focus on the animal. The majority of this time is spent automatically centring the animal within the field of view and subsequent focusing. The time reported for imaging includes the time required to capture the image, save it to the disk and switch back to the ×2 objective lens. Error bars show standard deviation. Figure 1: Design and characterization of the in-well cooling system. ( a–c ) In-well cooling device and its operation. ( a ) Individual cooling elements consist of an aluminium pin bonded to a thermoelectric cooler (TEC) with a copper pin bonded to the opposite side to dissipate heat. ( b ) Cooling elements can be arrayed to match various well configurations. ( c ) Pipelined cooling. Thermoelectrically cooled pins are inserted into wells containing animals. Once activated, a cooling element reduces the temperature of the well, immobilizing the animal(s) within that well. Immobilized animals are imaged or optically manipulated using inverted epifluoresence microscopy. Concurrently, neighbouring wells are cooled such that the animals to be subsequently imaged are immobilized in advance. ( d ) Temporal and spatial dependency of the temperature inside the well being cooled (near the sides and corners), in an orthogonally adjacent well (near the wall adjacent to the well being cooled, near the adjacent-well centre and near the side of adjacent well that is furthest from the well being cooled) and in a diagonally adjacent well (near the corner closest to the well being cooled). Thermoelectric cooling was started at t =0 s (first dashed line) and stopped at t =280 s (second dashed line). See Methods for measurement technique. ( e ) Time required for imaging animals inside a well plate with a single animal per well. Following imaging of the first animal in the well ( n =20), pipelined cooling enables much faster imaging of the subsequent animals ( n =95). The time reported for positioning/focusing includes the time required to move the position stage from well to well, locate an animal using a ×2 objective lens, switch to a ×20 objective lens and focus on the animal. The majority of this time is spent automatically centring the animal within the field of view and subsequent focusing. The time reported for imaging includes the time required to capture the image, save it to the disk and switch back to the ×2 objective lens. Error bars show standard deviation. Full size image Stable immobilization and imaging in multiwell plates During the low-temperature period, cellular-resolution fluorescence images of entire animals can be acquired ( Fig. 2a ). 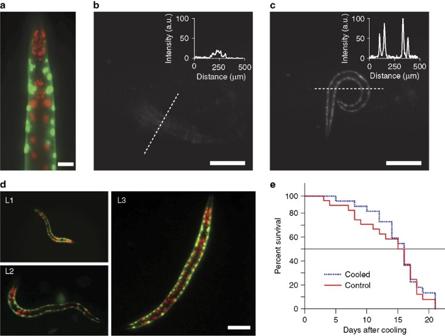Figure 2: In-well cooling enables immobilization and subcellular-resolution imaging ofC. elegansin standard multiwell plates. (a) Multichannel fluorescence image of an animal immobilized using in-well cooling. Green:his-72, red:unc-54 &pha-4. Scale bar, 30 μm. (b, c) Fluorescence image of an animal before and after cooling. (b) Before cooling, the animal is moving too rapidly for visualization at 10 frames s−1. (c) Following cooler activation, the animal's movement slows drastically allowing high-resolution imaging. Insets show fluorescence intensity across the section of the animal indicated by the dotted lines in each image. Cooling pin is visible on the right side of both images. Scale bar, 250 μm. (d) Immobilization of early-larval stageC. elegans. L1-L3 animals are immobilized with sufficient stability to image cellular features. Green:his-72, red:unc-54 &pha-4. Scale bar, 40 μm. (e) Effects on lifespan after cooling for 5 min every hour. There was no significant difference between the lifespans of the cooled (blue dashed line) and control (red solid line) populations (Logrank test;P=0.61). Figure 2b,c shows an animal before and after cooling and highlight the drastic improvement in image resolution. In addition to L4-stage and adult animals, this system can successfully immobilize early-larval stage animals ( Fig. 2d ). The reliability and reusability of this technology is very high because it does not use any moving parts or microfluidic components. Cycling a cooling element continuously for 25,000 cycles (1 min on, 30 s off) had no impact on the cooling performance ( Supplementary Fig. S2 ). This is equal to the number of cycles the system would perform if plates were imaged continuously at a rate of one plate per hour for 2.7 years. Figure 2: In-well cooling enables immobilization and subcellular-resolution imaging of C. elegans in standard multiwell plates. ( a ) Multichannel fluorescence image of an animal immobilized using in-well cooling. Green: his -72, red: unc -54 & pha -4. Scale bar, 30 μm. ( b, c ) Fluorescence image of an animal before and after cooling. ( b ) Before cooling, the animal is moving too rapidly for visualization at 10 frames s −1 . ( c ) Following cooler activation, the animal's movement slows drastically allowing high-resolution imaging. Insets show fluorescence intensity across the section of the animal indicated by the dotted lines in each image. Cooling pin is visible on the right side of both images. Scale bar, 250 μm. ( d ) Immobilization of early-larval stage C. elegans . L1-L3 animals are immobilized with sufficient stability to image cellular features. Green: his -72, red: unc -54 & pha -4. Scale bar, 40 μm. ( e ) Effects on lifespan after cooling for 5 min every hour. There was no significant difference between the lifespans of the cooled (blue dashed line) and control (red solid line) populations (Logrank test; P =0.61). Full size image In-well cooling does not affect animal health We recorded several measurements to assess how our technique influences animal physiology under frequent immobilization conditions. The difference between the lifespan of the repeatedly cooled animals (cooled for 5 min every hour for 24 h) and the lifespan of the control group ( Fig. 2e ) was nonsignificant (Logrank test; P =0.61). Similarly, repeated cooling did not affect the morphology of the animals nor their progeny count. Frequent cooling for time-lapse imaging also did not affect neurite regeneration, which is a highly dynamic process: Our technique enables the use of subcellular-resolution optical manipulation methods in multiwell plates, such as femtosecond laser microsurgery. Precise targeting of axons by a laser for microsurgery becomes possible when the animals are immobilized by cooling ( Fig. 3a ). Following surgery, axons regenerate ( Fig. 3b ) as we previously showed in the first observation of axonal regeneration in C. elegans [5] , [6] . We first determined whether cooling affects regeneration, by examining three different surgery conditions in young adult animals. We performed surgery both on anaesthetized animals on glass slides, and on animals immobilized using in-well cooling. After surgery, the animals axotomized under anaesthesia were split into two populations: one population recovered on agar plates and the other population recovered in a 96-well plate with liquid culture in the wells. Regeneration was observed 24 and 48 h following injury, and no significant difference was found between the regeneration observed in animals immobilized by in-well cooling and those immobilized by anaesthesia ( Fig. 3c ). We also examined whether frequent immobilizations following femtosecond laser microsurgery affect regeneration: There was no significant difference (Student's t -test; P =0.52) in the regeneration observed 48 h post surgery between a population that was cooled for 5 min every 6 h and a control population that was not cooled but was maintained under otherwise identical conditions ( Fig. 3d ). Repeated cooling similarly did not affect the regeneration of the olfactory amphid wing 'B' (AWB) neurons in the head (Student's t -test; P =0.33; Fig. 3d ). 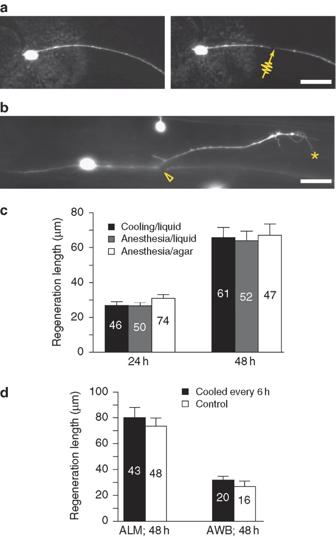Figure 3:In vivofemtosecond laser microsurgery in multiwell plates. (a) Localized ablation by femtosecond laser (seemethods) and (b) regeneration of anterior lateral mechanosensory (ALM) axon in mec-4::GFP animal. Arrow indicates point of surgery, triangle indicates starting point of regeneration and asterisk indicates end of maximum-length branch 48 h post surgery. Scale bars, 20 μm. (c) Effect of immobilization method and recovery conditions on regeneration following axotomy. Graph shows length of the longest regenerating branch from the cut point following axotomy of ALM neurons in young adult animals. There is no significant difference between the cooled (black bar) population and the anaesthetized control groups (grey bar for recovery in liquid, white bar for recovery in agar) either 24 h (Student'st-test;P=0.91 and 0.18 for the animals that recovered in liquid and on agar, respectively) or 48 h (Student'st-test;P=0.82 and 0.88, respectively) post surgery. The total number of animals in each experiment is indicated on the bar. (d) Effect of multiple immobilizations (every 6 h for 48 h) on regeneration of ALM and AWB neurons. There is no statistically significant difference between the regeneration measured in the cooled (black bars) and control (white bars) populations (Student'st-test;P=0.52 andP=0.33, respectively). The total number of animals in each experiment is indicated on the bar. Figure 3: In vivo femtosecond laser microsurgery in multiwell plates. ( a ) Localized ablation by femtosecond laser (see methods ) and ( b ) regeneration of anterior lateral mechanosensory (ALM) axon in mec-4::GFP animal. Arrow indicates point of surgery, triangle indicates starting point of regeneration and asterisk indicates end of maximum-length branch 48 h post surgery. Scale bars, 20 μm. ( c ) Effect of immobilization method and recovery conditions on regeneration following axotomy. Graph shows length of the longest regenerating branch from the cut point following axotomy of ALM neurons in young adult animals. There is no significant difference between the cooled (black bar) population and the anaesthetized control groups (grey bar for recovery in liquid, white bar for recovery in agar) either 24 h (Student's t -test; P =0.91 and 0.18 for the animals that recovered in liquid and on agar, respectively) or 48 h (Student's t -test; P =0.82 and 0.88, respectively) post surgery. The total number of animals in each experiment is indicated on the bar. ( d ) Effect of multiple immobilizations (every 6 h for 48 h) on regeneration of ALM and AWB neurons. There is no statistically significant difference between the regeneration measured in the cooled (black bars) and control (white bars) populations (Student's t -test; P =0.52 and P =0.33, respectively). The total number of animals in each experiment is indicated on the bar. Full size image Time-lapse imaging of in vivo neural regeneration Following surgery, we examined the axonal regeneration dynamics by frequently immobilizing and imaging several animals ( Fig. 4a and b ) over a 48-h time window. Analysis of single neurons showed that the majority of neurite regrowth (75±5.5%) occurs within a short 18-h window ( Fig. 4c ). In the absence of repeated single animal immobilization and imaging, only statistical averages can be obtained from end-point measurements on many animals. Such averaging (red dashed line in Fig. 4b,c ) underemphasizes the growth that occurs after the first 24 h post axotomy, obscuring that the period of largest growth in some instances can occur later ( Fig. 4d ). Use of the average regeneration rate also incorrectly predicts a significantly smaller amount of regrowth during any 18-h window (58 versus 75%, Student's t -test; P =0.008). 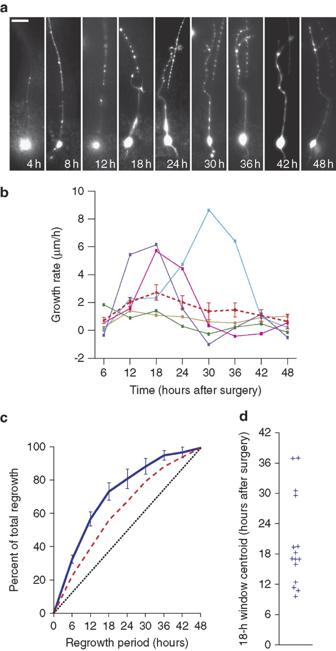Figure 4: Time-lapse imaging and analysis of neuronal regeneration dynamics in multiwell plates. (a) Time-lapse fluorescence images of a regenerating axon. Scale bar, 15 μm. (b) Representative curves of calculated growth rate of regenerating branch versus time. Each solid coloured line shows a measurement of the regrowth of a single neurite in an animal. Dashed red line shows mean growth rate averaged overn=15 animals. (c) Percentage of total regeneration occurring over a moving time window. Solid blue line shows the percentage of 48-h regeneration versus the time window calculated from multitime-point measurements on individual animals (n=15). Dashed red line shows the same calculation using the average growth rate measurements (red line inFig. 4b), and black dotted line shows the case if regeneration rate were constant. (d) Distribution of the centre of the 18-h window in which most of the regeneration occurs. All error bars are s.e.m. Figure 4: Time-lapse imaging and analysis of neuronal regeneration dynamics in multiwell plates. ( a ) Time-lapse fluorescence images of a regenerating axon. Scale bar, 15 μm. ( b ) Representative curves of calculated growth rate of regenerating branch versus time. Each solid coloured line shows a measurement of the regrowth of a single neurite in an animal. Dashed red line shows mean growth rate averaged over n =15 animals. ( c ) Percentage of total regeneration occurring over a moving time window. Solid blue line shows the percentage of 48-h regeneration versus the time window calculated from multitime-point measurements on individual animals ( n =15). Dashed red line shows the same calculation using the average growth rate measurements (red line in Fig. 4b ), and black dotted line shows the case if regeneration rate were constant. ( d ) Distribution of the centre of the 18-h window in which most of the regeneration occurs. All error bars are s.e.m. Full size image Performing screens entirely within multiwell plates confers several significant benefits. Because multiwell plates are commonly used, there already exists a wealth of equipment, robotics and protocols for screening in this format. As a result, our technology can expand the use of existing HTS systems to perform high-content multicellular organism screens at subcellular resolution. High-speed precise liquid handling equipment can be used to rapidly dispense precise volumes of screening compounds, and multiwell plates also simplify isolation of animals for multitime-point tracking of single animals throughout the experiments. Screening C. elegans entirely within multiwell plates also eliminates all the complexity, cost and unreliability associated with microfluidics, as well as the 'world-to-chip' fluidic interface issues for large-scale incubation of animals. Our cooling apparatus could be manipulated with high-throughput robotics, and also does not require any fluidic components; thus, it is not susceptible to clogging or loss of animals. No side effects on animal lifespan, neurite regrowth, progeny count or animal morphology are observed even after frequent immobilization and imaging of animals at multiple time points. Each well of a 96-well plate has sufficient volume of media to ensure that C. elegans is healthy over its entire lifespan, and 96-well plates were previously used to enable large-scale screening of C. elegans from L1 stage until death to identify chemicals that extend lifespan [21] . As C. elegans can produce significant numbers of progeny inside the wells, fluorodeoxyuridine is commonly used to induce sterility while still allowing animals to develop normally [21] , [22] , [23] . Absence of progeny simplifies tracking of animals throughout their entire lifespan, and reduces both the amount of feeding bacteria required and the buildup of waste inside the wells. Both forward and reverse genetic assays, as well as chemical assays, on C. elegans at subcellular resolution are possible in high-throughput-compatible multiwell plate formats using our technology. As is commonly done, animals can be dispensed into multiwell plates either by flow sorters [1] or by manual or automated liquid dispensers. Our device subsequently allows immobilization of animals in the individual wells for imaging at multiple time points. Forward genetic screens can be performed if mutagenized animals are dispensed into the wells. Reverse genetic screens or chemical screens can be performed if the animals are incubated in wells containing either chemicals or dsRNA-expressing bacteria. The pins can be sterilized either by commercial pin washers or via heating by running the TEC in reverse ( Supplementary Fig. S1 ). There are also a number of powerful image processing algorithms that, combined with our technology, can further enhance the ability to perform high-throughput and high-content screens on C. elegans . Using a low-magnification objective, an entire well can be imaged and the location of individual animals can be determined automatically [24] . Higher resolution images of individual animals can be automatically straightened in 3D [25] , which simplifies animal comparison and results in smaller file sizes. Automated cell-lineage tracing [26] , three-dimensional nuclei segmentation [27] and cell-body ablation [28] have all been demonstrated for C . elegans . Our work enables the use of these advanced image-processing techniques in an HTS-compatible format. C. elegans is a useful model for studying neuronal regeneration as its stereotypic anatomy and hermaphroditic reproduction allow repeated studies of the same type of neural injuries in isogenic animal populations, significantly enhancing the reproducibility of assays. Previous studies combining laser microsurgery and C. elegans have identified how several factors, including animal age, neuronal type, synaptic branching and axon guidance signalling, influence regeneration [29] , [30] , [31] . Laser microsurgery screens, as well as screens using nematodes exhibiting spontaneous neurite breaks due to dysfunction of β-spectrin, have also revealed that axon regrowth depends on the activity of MAP kinase pathways [31] , [32] , [33] . Most recently, we have demonstrated the use of microfluidics in combination with femtosecond laser microsurgery to perform chemical screens on neural regeneration in C. elegans [19] . This screen identified a role for protein kinase C in the regeneration of the posterior lateral mechanosensory (PLM) neurons following surgery and showed that the small molecule prostratin enhances regeneration. Our new in-well cooling technology can drastically scale up these investigations on neural degeneration and regeneration by using a format entirely compatible with existing HTS systems. In addition, time-lapse analysis can yield significant insight into many physiological processes that cannot be gained through end-point assays, as we illustrated here for neuronal regeneration following femtosecond laser microsurgery. Similarly, using our system to image and screen time-resolved expression patterns of many genes using fluorescent reporters such as elt-3:: GFP, ugt-9:: GFP and col-144:: GFP [34] can facilitate the study of the ageing process under variety of dietary, genetic and environmental conditions. Device construction and operation Individual cooling elements consist of a 6.6×6.6-mm TEC (NL1011T-01AC, Marlow Industries) and aluminium and coppers pins cut from ¼′' square rod. The aluminium pin is attached to the cooled surface of the TEC and the copper pin is attached to the opposite side of the TEC using a thermal adhesive (Arctic Alumina, Arctic Silver). A ¼′' thick copper backplane with ¼′' square holes cut into it is used to array the cooling elements and provide additional heat dissipation. The individual TECs are powered by a DC power supply set to 1.1 V (CS13005X III, Circuit Specialists), which draws a current of ∼ 0.6 A per active TEC. The entire device is placed in a 96-well plate with thin glass bottom (MGB096-1-2-LG-L, Matrical) so that wells can be imaged by a standard inverted epi-fluorescence microscope (Eclipse Ti-U, Nikon). Anti-fog drops (FogTech) are used to prevent condensation on the underside of the glass during cooling. Well temperature measurements Fine wire thermocouples (5TC-TT-T-40-36, Omega) were immersed into multiwell plates at various positions. Wells were filled with 150 μl of liquid nematode growth medium (NGM) and cooled using the described cooling technology. Thermocouple measurements were recorded using a temperature logger (HH147U, Omega). Nematode handling Nematodes were grown at 15 °C in NGM agar plates, unless otherwise stated. Standard procedures were followed for C. elegans maintenance [35] . Nematode strains used in this study included SD1726: Is[p his-72 GFP;p unc-54 H1::mCherry;p pha-4 mCherry], SK4005: zdIs5 [p mec-4 GFP]I and CX3553: lin-15B (n765) ky Is104 [p str-1 GFP]X. The first strain was a gift from the laboratory of Stuart Kim and the latter strains were obtained from the Caenorhaditis Genetics Center. Age synchronizations were performed by transferring ∼ 25 gravid adults to a fresh NGM agar plate and allowing them to lay eggs for 6 h at 20 °C. Following egg laying, the adults were removed and the plates were maintained at 15 °C for the animals to grow normally. Animals were loaded into the individual wells using a pick. Lifespan analysis Two populations of animals were incubated in 96-well plates, with six animals and 150 μl of liquid NGM supplemented with OP50 per well. The first population was cooled for 5 min every hour over a 24-h period and was maintained at room temperature for the remaining time. The control population was not cooled and was maintained at room temperature. Subsequently, both populations were transferred to agar plates with OP50 feeding bacteria in order to recover. Animals were observed once per day to assess mortality, and transferred to new plates when needed. Measurement of immobilization and image acquisition times Animals were incubated in 96-well plates with one animal per well in 100 μl of liquid NGM supplemented with OP50. The time required to immobilize and capture an image of an animal were recorded. The time reported for positioning/focusing includes the time required to move the position stage from well to well, locate an animal using a ×2/0.1 NA objective lens, switch to a ×20/0.75 NA objective lens and focus on the animal. The majority of this time was spent automatically centring the animal within the field of view and subsequent focusing. The time reported for imaging includes the time required to capture the image with 750-ms exposure, save it to the disk and switch back to the ×2 objective lens. For the first well of the plate, an additional time is required for the cooling to halt the movement of the animals because the first well does not benefit from the pipelined cooling ( Fig. 1c ). A Photometrics CoolSNAP HQ2 camera was used to acquire images. The field of view of this camera was 4.66×3.355 mm, using the ×2 objective lens. Laser surgery The optical path was set up as previously described [7] . To perform femtosecond laser microsurgery, a Mai-Tai HP (Spectra-Physics) femtosecond laser beam with 800-nm wavelength and 80-MHz repetition rate was delivered to the specimen by means of an inverted microscope (Eclipse Ti-U, Nikon). ALM and AWB axons were axotomized by pulses with 7-nJ energy for 1.5 ms, using a ×20/0.75 NA objective lens. For laser surgery on glass slides, synchronized nematodes were immobilized in 2% agarose pads with 10-mM NaN 3 . Measurements of axon regeneration were recorded and analyzed using a MATLAB program. Effects of immobilization methods on regeneration We performed surgery both on animals anaesthetized on agar pads, and on animals immobilized using in-well cooling. We cut one ALM axon per animal, 50 μm from the soma, using the laser parameters described above. Following surgery, we split the animals that were axotomized under anaesthesia into two populations, both maintained at 20 °C. One population recovered on agar plates whereas the other population recovered in a 96-well plate with six animals per well in 150 μl of liquid NGM supplemented with OP50. The animals that were axotomized using in-well cooling were maintained in a 96-well plate with six animals per well in 150 μl of liquid NGM supplemented with OP50. Regeneration length was measured either 24 or 48 h following injury. Effects of repeated immobilization on regeneration Surgeries were performed on young-adult animals 50 μm from the ALM soma or 30 μm from the AWB soma. Animals were immobilized by cooling in 96-well plates with six animals per well in 100 μl of liquid NGM supplemented with OP50. Following surgery, both populations recovered at 20 °C, although one population was also cooled for 5 min per well every 6 h. Regeneration length was measured 48 h post surgery. Multitime-point imaging and analysis Surgeries were performed on young adult animals 50 μm from the ALM soma. Animals were incubated in 96-well plates with 100 μl of liquid NGM supplemented with OP50 per well at 20 °C. The animals were immobilized by in-well cooling and imaged at multiple time points (4, 8, 12, 18, 24, 30, 36, 42 and 48 h post surgery). Regeneration length at 6 h was calculated by averaging data at 4 h and 8 h. Growth rates from 6–42 h were calculated from the regrowth length using a centre difference method and the 48-h growth rate was calculated using a backwards difference method. The centroids of the time windows were calculated as where v i is growth rate data from the time points t i that make up the time window. Statistical analysis Comparisons of regeneration lengths were performed using a two-tailed Student's t -test. Lifespan analysis was performed with the Logrank (Mantel-Cox) test using the GraphPad Prism software package. How to cite this article: Rohde, C.B. & Yanik M.F. Subcellular in vivo time-lapse imaging and optical manipulation of C. elegans in standard multiwell plates. Nat. Commun. 2:271 doi: 10.1038/ncomms1266 (2011).